Evidence for tactical concealment in a wild primate Theory predicts that cheating individuals should alter their behaviour to avoid detection, yet empirical data for such ‘deceptive’ behaviour (and its putative consequence—punishment) is almost entirely absent from the literature. This dearth of evidence, particularly among primates, limits our understanding of the evolution of deception and punishment. Here, we quantify deception and punishment in a reproductive context in wild geladas ( Theropithecus gelada ). Individuals involved in extra-pair copulations (9% of observed copulations) exhibited behaviour consistent with tactical deception: they were less likely to vocalize and more likely to copulate when the cuckolded male was a sizable distance away (>20 m). Further, many extra-pair copulations ( ∼ 20%) elicited post-copulatory aggression—likely, punishment—from cuckolded males. This rare empirical evidence of both tactical concealment and retaliatory aggression offers a potential model system for examining the co-occurrence of deception and punishment in natural settings. Sociality creates the potential for diverse behavioural strategies because animals both cooperate and compete with conspecifics. Defectors (in the case of cooperation) or subordinates (in the case of competition) may benefit from deceptive behaviour [1] , as deception may allow individuals to escape the social costs otherwise associated with cheating/cuckoldry (for example, [2] and [3] ). As such, there is considerable interest in identifying the factors that both favour and constrain deceptive behaviours. In animal studies, the most widely used definition of deception is ‘tactical deception’; that is, an actor employs a signal or action in an atypical context, thereby disadvantaging a misinformed competitor, to the benefit of the actor [4] , [5] . This flexible use of behaviour includes the active falsification of signals and the withholding of specific signals [5] , [6] . Current evidence for tactical deception comes primarily from either anecdotal reports or captive studies across several taxa [7] , [8] , [9] , [10] , with rather limited empirical evidence coming from wild/free-ranging populations [11] , [12] , [13] . It has been argued that that large-brained, highly social primates may be particularly adept at deception [9] , [14] . Additionally, some primates have demonstrated the ability to understand the visual perspective of a rival in competitive contexts [15] , [16] , [17] , suggesting that sophisticated forms of deception may be a possibility. In a classic example of this, rhesus macaques ( Macaca mulatta ) were reported to deceptively withhold food calls and, if discovered, received punishment [18] . However, this case has since been reinterpreted: rather than withholding food calls, monkeys may have been failing to ‘claim’ the food item and thus (if discovered) aggressive competition for the item ensued [19] (see also [20] for a similar argument in white-faced capuchins, Cebus capucinus ). If this singular case is removed from the roster of evidence for primate tactical deception, the evidence supporting such behaviour is reduced to anecdotes from the wild and reports from captive studies (with one possible exception of ‘functional’ deception in the context of food competition [21] ). Moreover, at least one study on a wild primate reports a lack of tactical deception in a context (that is, sneak copulations), where it would presumably benefit a subordinate male [22] . Certainly, evidence for tactical deception is difficult to document in wild primates where experimental manipulations can be challenging. Consequently, the question arises as to whether this constitutes an absence-of-evidence or rather evidence-of-absence for tactical deception in wild primates. Punishment is a behavioural strategy that may curtail cheating/cuckoldry. Punishment occurs when an individual responds to a (perceived) reduction in his fitness by inflicting negative consequences on the perpetrator(s), without gaining an immediate fitness benefit [19] , [23] , [24] . A delayed benefit to the punisher is expected in the form of future behavioural modification (that is, cooperation) in the punished parties [19] , [23] , [24] . Models of human [24] , [25] and non-human animal cooperation [19] , [23] , [26] assume that punishment has evolved, in part, due to the delayed benefit of future cooperation in the punished individuals. However, punishment is rarely observed outside the context of human society [27] , mainly because most intraspecific aggression results in an immediate benefit for the aggressor, thereby qualifying as a form of direct competition [19] , [26] . A few studies have explicitly demonstrated the punishment of non-cooperative behaviour in birds [2] and fish [28] , but its scarcity in primates is surprising given the importance of punishment in human societies [25] , [27] . Further, punishment seldom leads to clear behavioural modifications (that is, increased cooperation or decreased competition) in the punished parties [29] , and there is some debate about the importance of behavioural modification in the evolution of punishment [30] . The limited evidence for the existence of both deception and punishment in the wild, particularly among primates, impairs our evolutionary understanding of cooperative and competitive strategies. Competition for mates is ubiquitous and has dramatic fitness consequences, making it a likely arena for observing sophisticated behavioural strategies such as deception and punishment. Here, we examined the mating behaviour of a wild primate with known levels of extra-pair paternity [31] . Male geladas, Theropithecus gelada , obtain reproductive success by becoming the dominant ‘leader’ male of a reproductive unit comprising 1–12 adult females (hereafter, ‘unit’). Typically, males gain dominance through aggressive takeovers [32] , although other avenues have been suggested [33] . Although these units aggregate into large, highly concentrated herds that provide ample opportunity for extra-pair copulation (EPC) [34] , extra-unit paternity has never been documented [31] . However, some units have 1–5 subordinate ‘follower’ males that sire a small percentage (17%) of the unit’s offspring [31] . Despite taking away some reproduction from the leader male, follower males provide a net benefit to leaders through shared unit defence, and thus a longer tenure for the leader [31] . Although aggression between these males is typically very low [35] , there is likely to be conflict over the amount of reproduction that followers gain (similar to many social vertebrates [36] and invertebrates [37] ), creating an incentive for concealed extra-pair copulations (EPCs; which, in this case, only refers to copulations involving followers males and unit females, and not extra-unit copulation s ). The high genetic stakes associated with reproduction by subordinates (common across a range of taxa [38] , [39] , [40] ) may create strong incentives for deception (for subordinate males) and punishment (for dominant males). The loud vocalizations that typically accompany gelada copulations [41] , [42] , combined with the open grassland habitat where concealment is difficult, suggest that EPCs should be easily detectible unless the individuals involved in the EPC (that is, the cuckolders) modify the usual gelada copulatory behaviour. Thus, theory suggests that cuckolders should exhibit deceptive behaviour to avoid receiving punishment from dominant males. We used long-term observational data from a population of wild geladas to assess the principal hypothesis that geladas employ deception and punishment to maximize their own reproductive success. Four predictions stem from this hypothesis: males and females will be less likely to vocalize during EPCs compared with within-pair copulations (WPCs, which include any copulation between a dominant male and one of his unit females); cuckolders will flexibly alter their behaviour, depending on the location of the cuckolded leader male; leader males will exhibit aggression towards individuals that are discovered during an EPC; recipients of aggression will not commit additional EPCs after receiving ‘punishment’. Distinctions between within-pair and extra-pair copulations The majority of copulations were WPCs (90.99%; 939/1,032) and most were accompanied by vocalizations from one or both individuals (90.02%; 929/1,032). In observed EPCs, we found evidence for vocal suppression: both sexes were more likely to vocalize during WPCs than EPCs ( Fig. 1a ; female vocalization model WPC estimate±s.e.m.=1.31±0.61, z -score=2.14, P =0.032; Fig. 1b : male vocalization model WPC estimate±s.e.m.=1.72±0.60; z -score=2.87, P =0.004). In a within-subjects analysis, this pattern was also reflected in the three cases where follower males were former leader males that had lost their leadership position: as leaders, these males vocalized in 15/15 copulations; as followers, they vocalized in 4/10 copulations (binomial test of proportions: 95% confidence interval=0.21–0.99, P= 0.019). Further, a generalized linear mixed model (GLMM) revealed a significant interaction between unit stability and male status for both male and female copulation calls. Although both sexes were more likely to vocalize for WPCs compared with EPCs during the stable period, this was not true for the unstable period ( Fig. 1a ; copulation type × stability estimate±s.e.m. for females=1.44±0.76, z -score=1.90, P= 0.058; Fig. 1b : males=1.52±0.73, z -score=2.07, P= 0.038). However, the stability of the time period by itself did not influence the likelihood of female (stability estimate±s.e.m.=−0.30±0.61, z -score=−0.49, P= 0.625) or male (stability estimate±s.e.m.=−0.22±0.57, z -score=−0.38, P= 0.704) vocalizations. 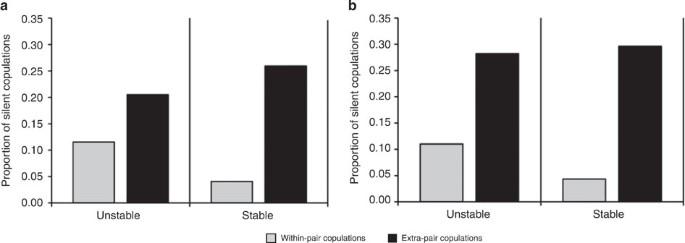Figure 1: Non-vocal copulations. The proportion of copulations in which (a) the female, and (b) the male remains silent. During the stable and unstable period, both sexes were significantly more likely to remain silent when engaged in an extra-pair copulation. (n=54 extra-pair copulations and 367 within-pair copulations during stable period;n=39 extra-pair copulations and 572 within-paircopulations during unstable period). Figure 1: Non-vocal copulations. The proportion of copulations in which ( a ) the female, and ( b ) the male remains silent. During the stable and unstable period, both sexes were significantly more likely to remain silent when engaged in an extra-pair copulation. ( n =54 extra-pair copulations and 367 within-pair copulations during stable period; n =39 extra-pair copulations and 572 within-paircopulations during unstable period). Full size image Analysis of female vocal behaviour suggests that female reproductive state was not the primary determinant of variation in vocal behaviour. Sixteen females copulated with multiple partners (both leader and non-leader males) on a single day ( n =18 days, comprising n =33 WPCs and 28 EPCs). Consistent with the data from all copulations, females were less likely to vocalize during these EPCs (WPC estimate±s.e.m.=2.55±1.10, z -score=2.32, P= 0.020). A subset of the copulation data indicates that EPCs were more likely to occur than expected when leader males were >20 m away from the copulating pair ( Fig. 2 ; χ 2 goodness-of-fit test: χ 2 =67.29, df=3, P <0.001). This is notable as leader males and followers spend <6% of the time at this distance ( Fig. 2 )—generally they are found closer together. In contrast to EPCs, WPCs did not deviate from expected distances between leader and follower males ( Fig. 2 ; χ 2 =6.84, df=3, P= 0.077). Both sexes reduced the percentage of silent copulations as the distance to leader male increased ( Fig. 3 ; males: χ 2 =74.75, df=3, P <0.001; females: χ 2 =60.21, df=3, P <0.001). However, these results have to be treated with caution as sample sizes were small and data were not fully independent (some individuals were represented twice in the data set). 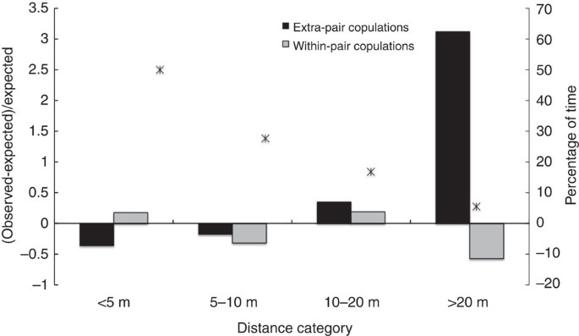Figure 2: Copulations at different male–male distances. The frequencies with which copulations occurred at various distances between the leader and follower male. The ‘expected’ frequency of occurrence is based on the amount of time leaders and followers typically spend at various distances from one another. Extra-pair copulations do not adhere to these predicted frequencies, but occur significantly more often when leader males are >20 m away from the copulating pair (see text for details). Asterisks indicate the percentage of time that leader and follower males spend at specified distances apart. (n=25 extra-pair copulations,n=85 within-pair copulations). Figure 2: Copulations at different male–male distances. The frequencies with which copulations occurred at various distances between the leader and follower male. The ‘expected’ frequency of occurrence is based on the amount of time leaders and followers typically spend at various distances from one another. Extra-pair copulations do not adhere to these predicted frequencies, but occur significantly more often when leader males are >20 m away from the copulating pair (see text for details). Asterisks indicate the percentage of time that leader and follower males spend at specified distances apart. ( n =25 extra-pair copulations, n =85 within-pair copulations). 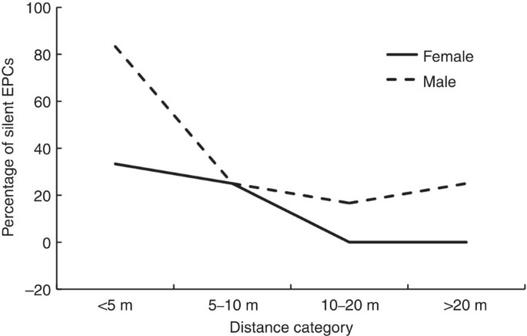Figure 3: Silent cuckoldry related to male–male distance. The percentage of EPCs in which males and females did not vocalize, at different distances between leader and follower male. (n=20 EPCs). Full size image Figure 3: Silent cuckoldry related to male–male distance. The percentage of EPCs in which males and females did not vocalize, at different distances between leader and follower male. ( n =20 EPCs). Full size image Retaliatory aggression We identified 17 aggressive acts that occurred within 5 min after an EPC (that is, 18.28% of all EPCs). This is a significant increase in rate of aggression received (2.19 acts per h), compared with baseline aggression received on days without EPCs (0.04 acts per h; Fisher’s exact test: P= 0.004). Compared with the overall percentage of silent EPCs (11.83%), cuckolders that received aggression were relatively silent: both individuals were silent in 35.29% of punished copulations. Few attacks were followed by copulation: only one leader male mated with the female within 5 min of attacking the cuckolding male, whereas none of the punished individuals engaged in another EPC within this same time period. All but one cuckolder (a female) were observed in EPCs on later dates. This is the first study to systematically document tactical deception in a primate living in a natural environment. In agreement with our first two predictions, follower males and unit females flexibly suppressed the copulation vocalizations typical of within-pair copulations, and paid close attention to the position of the leader male. Although withholding information is considered a ‘simpler’ form of deception than the active falsification of signals [5] , [43] , this ‘audience effect’ [44] , [45] on gelada copulation vocalizations suggests that their reproductive concealment may be tactical [46] . In contrast to rhesus macaques [22] , where subordinate males spend the majority of time on the periphery of social groups, geladas appear to strategically tailor their behaviour to take into account variability in the risk of detection, that is, their distance to the dominant male. The evidence for punishment was less clear. Following our third prediction, retaliatory aggression increased after EPCs compared with baseline aggression levels, with nearly 20% of all EPCs leading to attacks from leader males. Such attacks were aggressive responses to a potential fitness reduction, and thus follow the pattern of ‘negative reciprocity’ that characterizes functional punishment [19] , [23] . Moreover, we failed to find any immediate benefit gained by the punishers. Leader males did not generally copulate with the female immediately after attacking the cheaters, allowing us to rule out the possibility that the aggression was simply conflict over access to receptive females [19] . However, in contrast to our last prediction, punishers also did not gain delayed benefits—the majority of cuckolders did so again in the weeks and months after receiving punishment. Our study therefore provides support for a relatively recent idea in the debate about the function and evolution of punishment [30] : punishers may benefit from the act even if punished individuals do not modify their subsequent behaviour. Nakao and Machery [30] suggest that punishment in vertebrates may be a cost-cutting (minimizing harm to the punisher) or a cost-imposing (making the initial behaviour costly for the punished individual) strategy rather than a method of changing the future behaviour of the cheater/cuckolder. However, if the benefits of ‘punishment’ are immediate (as some cost-cutting behaviours appear to be), this raises the issue of how to differentiate punishment [19] from other forms of competition. Further data from wild populations are needed to better understand the costs and benefits of punishment-like behaviours. Similar to other primates [47] , these results suggest that gelada copulation calls are not an incidental by-product of the sexual act, but rather are under voluntary control. Gelada copulation calls exhibit an audience effect, similar to alarm and food calls in many species (for example, [44] , [45] and [48] ). However, the function of gelada copulation calls remains unclear, especially when considering that call function is likely to be sexually dimorphic. In many species, female copulation calls incite male–male competition [49] . By contrast, we found limited evidence of post-copulatory competition in geladas (see also [50] ), and the most highly motivated adult males (bachelors) frequently ignore copulation vocalizations altogether [41] . Male copulation calls may be a potential indicator of ejaculation [42] , but we found no indication that ejaculation was absent in silent copulations. Alternatively, both sexes’ copulation calls may indicate fertility and rank [51] , [52] or function to strengthen the pair bond between the partners [47] , [53] , as they occur during—not after—mounting and ejaculation. The clear flexibility in vocal behaviour depending on distance to the leader male suggests, however, that vocalization rates do not simply decrease with a low-ranked partner or between individuals with weak social bonds (that is, the follower and unit females [35] ). Additionally, the acoustic properties of copulation calls themselves may be indicative of social status, similar to those of other primates [51] , [52] . Experimental work is needed to fully understand the function of copulation calls in geladas. Geladas’ social knowledge in their large, fluid societies has been shown to be limited: males do not know the identities of, or relationships between, individuals outside their immediate reproductive unit or all-male (bachelor) group [41] , [54] . However, the occurrence of punishment and deceptive behaviour gives us the opportunity to investigate other cognitive skills, such as temporal discounting and higher order intentionality [55] , [56] (that is, awareness of the mental state of the individuals they are deceiving). For example, the tactical concealment shown here suggests that geladas (in this case, the cuckolders) may account for the visual and acoustic perspective of others [16] , [57] . Alternatively, however, the occurrence of punishment creates the potential for a less sophisticated cognitive mechanism at work—mainly, that cuckolders acquire deceptive behaviour through associative learning [4] . Thus, in addition to increasing our understanding of the costs and benefits of different behavioural strategies, the presence of deception and punishment in geladas allows us to further assess the cognitive underpinnings of their social behaviour. Ethical note This research was approved by the University Committee on Use and Care of Animals (UCUCA) at the University of Michigan and adhered to the laws and guidelines of Ethiopia. Study site and subjects All research was conducted on a population of geladas living in the Simien Mountains National Park, Ethiopia, where a subset of individuals has been under continuous observation since January 2006. We collected observations on adult males ( n =73) and females ( n =134) in 19 reproductive units from January 2009 to December 2011, constituting 2600, h of observational data. Data collection included the following: (1) 15-min focal animal samples [58] where observers noted all behaviours of the focal individual; (2) distances between the focal animal and other group members at 5-min intervals within each focal animal sample; (3) scan samples at 20-min intervals to establish the distances between dominant leaders and subordinate followers, with inter-individual distances categorized as: <5 m, 5–10 m, 10–20 m and>20 m apart; and (4) all occurrences of agonistic and sexual behaviour within a selected unit for 2–3 h at a time. This data collection protocol ensured that most (if not all) copulations were noted, although we acknowledge that there may be an observational bias towards loud, conspicuous copulations. Across the study, each unit experienced one or more takeovers—that is, when a challenger male replaced the leader male. Takeovers are highly disruptive events, typically involving multiple bachelor males harassing the leader male until he is ousted from the leadership position by one of them. For up to 3 months after the takeover, units are more vulnerable to unit fissions (that is, the permanent breakup of a unit into smaller, socially discrete units) and experience elevated rates of fighting and EPCs [41] . Typically, such units are found in closer proximity to bachelors and contain additional, temporary follower males [41] as compared with units outside this unstable period. To assess variation in copulatory or aggressive behaviours between these periods, we separated our observations into ‘unstable’ (<90 days after a takeover) and ‘stable’ (>90 days after the most recent takeover) periods. Distinctions between within-pair and extra-pair copulations Gelada copulations are typically accompanied by loud, individually distinct vocalizations uttered by both the male and female partner [41] . We categorized each copulation event as either a WPC (involving a leader male) or EPC (involving a follower male). For each copulation, we noted which individuals emitted copulation vocalizations. We then used binomial GLMMs with a logit link function to examine the effect of male status (leader or non-leader), the stability of unit (stable or unstable) and the interaction between these two fixed effects on vocalization production during copulation. The identity of the male and females were entered as random effects. We fit one GLMM for each of the two binary outcome variables: (1) female vocalized or was silent, and (2) male vocalized or was silent. These analyses were conducted using the lme4 package in R Statistics [59] . Because female primates’ copulation vocalizations may vary with the phases of their oestrous cycles [51] , we attempted to control for the possible influence of reproductive state on female geladas’ vocal behaviour. In the absence of complete hormonal records for all females within this dataset, we controlled for oestrous state by examining the vocal behaviour of females that mated with multiple males on any given day. If the female’s vocal behaviour varied with her reproductive state, we would expect her to be consistently silent or vocal on these days, irrespective of the male with which she mated. For all females, we therefore identified the days on which they engaged in both WPC and EPC, and compared their vocal behaviour using binomial GLMs. Finally, to gauge whether or not deception was tactical, we assessed the social context in which EPCs occurred. Using leader–follower distance data from scan samples ( n= 1088 data points for units with followers), we determined the expected distances between leaders and followers within our population. Subsequently, we extracted all copulations from all-occurrence ( n= 92) and focal data ( n =15) that were noted within 5 min of such a distance data point. We then calculated how many EPCs ( n =22 events) and WPCs ( n =85 events) occurred within each leader–follower male distance category. We compared these observed numbers with the expected numbers using χ 2 goodness-of-fit tests. Finally, we assessed the flexibility of vocal behaviour during EPCs by calculating the proportion of copulations in which males and females were silent across four distance categories. We compared these proportions to a random distribution of silent copulations. Retaliatory aggression To examine putative punishment of EPC in geladas, we noted aggression by leader males towards the cuckolders. We scored aggression by the leader male in the 5 min following each EPC, noting all chases and biting attacks directed at the copulating pair. Using a binomial test of proportions, we compared these observed rates of aggression with expected rates of aggression, calculated from 76.75 h of focal data on follower males on days without EPCs. Additionally, whenever we observed an attack following an EPC, we noted whether or not the attacker (leader male) copulated with the female within a 5-min period after the attack, which may be a sign of overt reproductive competition instead of punishment (a common consequence of primate copulations [49] ). How to cite this article: le Roux, A. et al. Evidence for tactical concealment in a wild primate. Nat. Commun. 4:1462 doi: 10.1038/ncomms2468 (2013).